Stepwise histone modifications are mediated by multiple enzymes that rapidly associate with nascent DNA during replication The mechanism of epigenetic inheritance following DNA replication may involve dissociation of chromosomal proteins from parental DNA and reassembly on daughter strands in a specific order. Here we investigated the behaviour of different types of chromosomal proteins using newly developed methods that allow assessment of the assembly of proteins during DNA replication. Unexpectedly, most chromatin-modifying proteins tested, including methylases, demethylases, acetyltransferases and a deacetylase, are found in close proximity to PCNA or associate with short nascent DNA. Histone modifications occur in a temporal order following DNA replication, mediated by complex activities of different enzymes. In contrast, components of several major nucleosome-remodelling complexes are dissociated from parental DNA, and are later recruited to nascent DNA following replication. Epigenetic inheritance of gene expression patterns may require many aspects of chromatin structure to remain in close proximity to the replication complex followed by reassembly on nascent DNA shortly after replication. Currently, it is not known how the status of gene expression is propagated through S and M phases when major changes to chromatin architecture occur. Re-establishment of parental chromatin structure on nascent DNA of future daughter cells in S phase may occur by a two-step mechanism in which most proteins and nucleosomes dissociate from DNA [1] , but a few molecules can quickly re-associate with DNA following replication. Such proteins or modifications may have an epigenetic role if they mark specific regulatory DNA sequences and then trigger association of the rest of the components of chromatin, probably in a specific order. This would lead to re-establishment of chromatin environment in the regulatory regions of the genes, and allow reconstitution of the gene expression status in daughter cell [2] , [3] . Until recently, this model of chromatin assembly remained untested in vivo , because there were no experimental approaches to examine the behaviour of chromosomal proteins other than histones at the time of, and shortly after the passage of the DNA replication complex in vivo . We recently developed several in vivo approaches to examine the proximity of chromosomal proteins to PCNA during replication and at the time of their recruitment to nascent DNA following replication [4] . Using these new tools in Drosophila embryos, we found that TrxG and PcG proteins TRX and E(z), H3K4 and H3K27 histone-methyltrasferases (HMTs), respectively, and PC, a component of the PRC1 complex, associate with their response elements (TREs and PREs) during DNA replication in vivo [4] . These results are in agreement with a previous study showing that several components of the PRC1 complex are stably bound to DNA in the in vitro replication assays [5] , [6] , and that these proteins are associated in vivo with relatively short stretches of nascent DNA [5] . Surprisingly, H3K4me3 and H3K27me3 are not detected in proximity to PCNA or nascent daughter strands of DNA, and initial accumulation of these methyl marks on H3 was detected only following S phase [4] . Together, these studies suggest that some TrxG and PcG proteins may function to re-establish active or repressing chromatin environments due to their ability to remain in close proximity to PCNA, or be rapidly recruited to nascent DNA following replication. These findings raise three essential questions: First, can other chromosomal proteins remain in proximity to PCNA or on nascent DNA following replication? Second, why are some histone modifications delayed despite the early presence of histone-modifying enzymes on nascent DNA? Third, what is the order of recruitment of chromosomal proteins to daughter DNA after replication? These issues are particularly important for proteins that are involved in changing the structure of chromatin, some of which are characterized genetically as members of the TrxG and PcG of epigenetic regulators [7] , [8] , but also include other chromatin modifiers or nucleosome remodelers. In this study we show that most chromatin-modifying enzymes, but not subunits of chromatin-remodelling complexes, are found in close proximity to PCNA and nascent DNA shortly after DNA replication. We conclude that epigenetic inheritance of gene expression patterns requires that multiple molecules remain in close proximity to the replication complex. Examining post-replicative protein assembly by PLA and CAA To address these questions, we used two assays to survey the behaviour of several groups of histone-modifying and nucleosome remodelling proteins during DNA replication in Drosophila embryos. To examine whether tested proteins are in close proximity to PCNA in the DNA replication complex or bound to DNA following replication we used the Proximity Ligation Assay (PLA, Olink, Bioscience). The results of PLA were found previously to be in excellent correlation with physical association of TRX, E(z) and PC, with the same DNA fragments as PCNA as detected in sequential re-ChIP assays [4] . Extensive characterization of these re-ChIP assays revealed that these proteins bind to their specific binding DNA sites, TREs and PREs, during or immediately following DNA replication [4] , validating the PLA assays with PCNA as a reliable source of information not only for transient presence of these proteins in close proximity to the DNA replication complex but also for their association or close proximity to DNA during the passage of the replication complex. It should be noted that PLA is a very sensitive technique with a dynamic range that detects proximity of single molecules (Olink), and thus can detect very rare and transient interactions. For comparison, TRX and PC interactions with PCNA are easily detectable by PLA [4] , but we were not able to detect these interactions in co-immunoprecipitation experiments ( Supplementary Fig. S1 ). We also used a recently developed Chromatin Assembly Assay (CAA) that is based on labelling of nascent DNA with EdU that is subsequently chemically conjugated with biotin. The antibodies to the tested protein and biotin are then used in a PLA assay to examine proximity of this protein to nascent DNA [4] . The shortest time for reliable EdU labelling in Drosophila embryos is 4–5 min. With an average speed of DNA replication of about 40 bp per sec, and considering that EdU entering into the nucleus may require some time, 4–5 min of EdU labelling will detect less than 10 kb of nascent DNA. Previously, we showed that the results of CAA correlate completely with the results of re-ChIP and PLA assays with PCNA [4] . The results of this and our previous study show that all proteins that are in close proximity to PCNA are also detected in the CAA assays after 4–5 min of EdU labelling. Proteins that are not detected in these two assays are always detected after longer times of EdU labelling. Thus, simultaneous use of two complementary assays, PLA and CAA, provide a means to survey for proximity to PCNA and time of recruitment of many proteins to nascent DNA at many genomic locations. Re-ChIP assays are not practical for testing multiple proteins because they require prior identification of binding sites at specific targets and large amounts of well-characterized specific antibodies that are not always available from commercial or other sources. Association of ASH1 and SET1 HMTs with replicating DNA The HMTs E(z) and TRX are in close proximity to PCNA and nascent DNA [4] . E(z) is the only H3K27 HMT in Drosophila . There are, however, several other H3K4 HMTs in addition to TRX, including ASH1 and dSET1. These proteins belong to different families of HMTs, and have different contributions to the overall levels of methylated H3K4 forms in different tissues [9] , [10] . Similar to TRX, dSET1 is in close proximity to PCNA ( Fig. 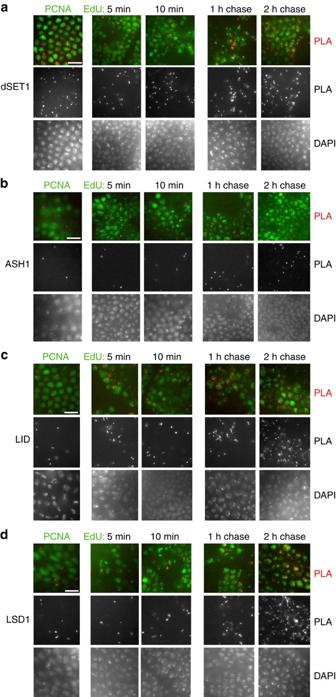Figure 1: Proximity of H3K4 HMTs and de-HMTs to PCNA and nascent DNA inDrosophilaembryos. (a–d) Proximity of H3K4 HMTs dSET1 (a) and ASH1 (b), and proximity of H3K4 de-HMTs LID (c) and LSD1 (d) to PCNA (left columns) and nascent DNA (columns 2–5) in gastrulatingDrosophilaembryos. Columns 2, 3, PLA with DNA labelled with EdU for 5 and 10 min. Columns 4, 5, DNA was pulse labelled with EdU for 10 min and chased for 1 and 2 h. PLA signals are in red. PLA signals from the same images are shown in the middle panels. DAPI staining of DNA of the same images are shown in the bottom rows. The results are from three independent experiments. Scale bar, 10 μm. 1a ; all the results on proximity of different proteins to PCNA and nascent DNA are summarized in Table 1 ). In CAA experiments, dSET1 is in proximity to nascent DNA labelled with EdU for 5 min. Its amount is slightly increased from 10 min to 2 h of EdU incorporation. Contrary to TRX and dSET1, ASH1 is not found in proximity to PCNA in the PLA assay ( Fig. 1b ). Consistent with this, ASH1 is not detected by CAA on nascent DNA until 1 h labelling with EdU, and its amount is slightly increased at 2 h of EdU incorporation. The occasional PLA signals that are seen with ASH1 in columns 1–3 (and in some figures below) do not overlap with PCNA- and EdU-labelled nuclei, and represent a typical low antibody background in the control experiments when only one of the tested antibodies is used for the PLA reaction [4] . In the gastrulating Drosophila embryos shown in this figure, the G1 phase is not detectable, S phase is about 50 min, and most transcription occurs in a G2 phase of variable length that depends on cell type [11] . Thus, ASH1 may be recruited either during mid-S phase or transcriptional G2 interphase. These results suggest that ASH1 may not be required for maturation of chromatin immediately after replication, potentially because it has cell cycle stage-specific activity. Figure 1: Proximity of H3K4 HMTs and de-HMTs to PCNA and nascent DNA in Drosophila embryos. ( a – d ) Proximity of H3K4 HMTs dSET1 ( a ) and ASH1 ( b ), and proximity of H3K4 de-HMTs LID ( c ) and LSD1 ( d ) to PCNA (left columns) and nascent DNA (columns 2–5) in gastrulating Drosophila embryos. Columns 2, 3, PLA with DNA labelled with EdU for 5 and 10 min. Columns 4, 5, DNA was pulse labelled with EdU for 10 min and chased for 1 and 2 h. PLA signals are in red. PLA signals from the same images are shown in the middle panels. DAPI staining of DNA of the same images are shown in the bottom rows. The results are from three independent experiments. Scale bar, 10 μm. Full size image Table 1 Proximity of chromosomal proteins and modified histones with PCNA and nascent DNA Full size table The presence of TRX and dSET1 on nascent DNA in the absence of H3K4me3 (ref. 4 ) suggests that the H3K4 tri-methylation activity of these HMTs is delayed following replication. As these enzymes are also mono- and di-methylate H3K4 to different extents [10] , it is possible that H3K4me1 and H3K4me2 appear earlier than H3K4me3 after DNA replication. However, similar to H3K4me3 (ref. 4 ), H3K4me2 and H3K4me1 are not detected in the proximity to PCNA and are detected on nascent DNA only at about 1 h after DNA replication, with the subsequent increase after 2 h of chase following EdU incorporation ( Fig. 2 and Table 1 ). 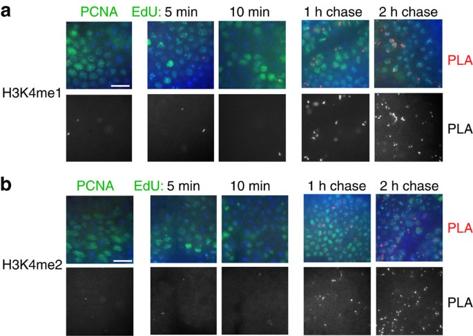Figure 2: Proximity of H3K4me1 and H3K4me2 to PCNA and nascent DNA. Antibodies against H3K4me1 (a) and H3K4me2 (b) were used for PLA with PCNA (left column) and for CAA with EdU-labelled DNA (columns 2–5). Both histone H3 forms are first detected on DNA labeled with EdU for 1 h. The results are from four independent experiments. Scale bar, 10 μm. Figure 2: Proximity of H3K4me1 and H3K4me2 to PCNA and nascent DNA. Antibodies against H3K4me1 ( a ) and H3K4me2 ( b ) were used for PLA with PCNA (left column) and for CAA with EdU-labelled DNA (columns 2–5). Both histone H3 forms are first detected on DNA labeled with EdU for 1 h. The results are from four independent experiments. Scale bar, 10 μm. Full size image UTX and CBP mask the activity of E(z) following replication The preceding results suggest that the activity of HMTs may be masked by the stronger activities of the lysine demethylases that are in proximity to nascent DNA immediately after replication and during S phase. Therefore, we examined the behaviour of two H3K4 demethylases during DNA replication. Drosophila Lid (ortholog of the mammalian Rbp-2/JARID1A and Plu-1/JARID1B) and Lsd1 are demethylases with overlapping H3K4me1/2 and H3K4me2/3 activities, respectively [12] , [13] , [14] , [15] . Both demethylases are found in proximity to PCNA and to nascent DNA labelled with EdU for 5 min ( Fig. 1c,d ). The simultaneous presence and presumably stronger activities of demethylases may preclude methylation of H3K4 by HMTs until the relative activities of these antagonistic enzymes change at some time after DNA replication. It is difficult to test this idea for H3K4 given the large number of potentially redundant H3K4 HMTs and demethylases. However, for H3K27, only one HMT and one demethylase with this specificity are present in Drosophila. We have shown previously that H3K27 HMT E(z) is in proximity to nascent DNA after 5 min of EdU labelling, but H3K27me3 is detected only after 1 h following labelling [4] . UTX is an H3K27me2/3 demethylase, an ortholog of the mammalian UTX, UTY and JmjD3 (ref. 16 ). As UTX is also found in proximity to PCNA and nascent DNA early after DNA replication ( Fig. 3a ), we tested the possibility that the demethylating activity of UTX may prevent H3K27me3 accumulation on nascent DNA at early stages following DNA replication. Inhibition of the UTX activity with the recently described compound GSK J4 (ref. 17 ) leads to the emergence of a considerable number of PLA signals in the CAA assay between H3K27me3 and nascent DNA labelled for EdU for 15 min, whereas non-treated embryos show no PLA signals ( Fig. 3d ). 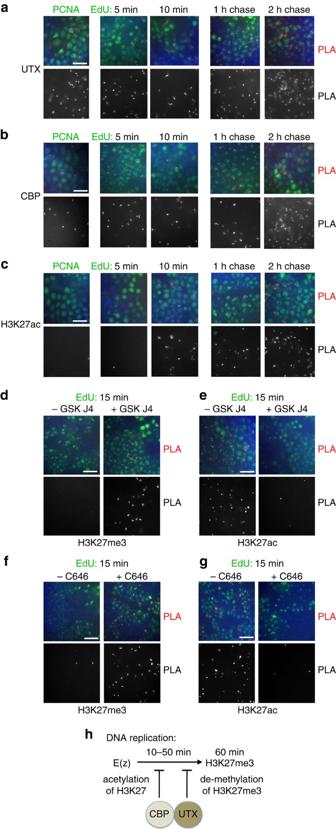Figure 3: Acetylation of H3K27 by CBP and demethylation of H3K27 by UTX may prevent methylation of H3K27 by E(z). (a) Proximity of H3K27 de-HMT UTX, HAT CBP and H3K27ac to PCNA and nascent DNA. (b,c) Inhibition of UTX activity by GSK J4 (b) and CBP activity by C646 (c) leads to early accumulation of H3K27me3 (left) and loss of H3K27ac (right). Embryos were incubated with (left columns) or without (right columns) GSK J4 (b) or C646 (c). They were then labelled with EdU for 15 min, followed by the PLA between biotin and either H3K27me3 or H3K27ac. Following CAA, embryos were immunostained for biotin (EdU, in green). (d) A scheme of proposed inhibition of H3K27 methylation by E(z) by CBP and UTX following DNA replication. The results are from four independent experiments. Scale bar, 10 μm. Figure 3: Acetylation of H3K27 by CBP and demethylation of H3K27 by UTX may prevent methylation of H3K27 by E(z). ( a ) Proximity of H3K27 de-HMT UTX, HAT CBP and H3K27ac to PCNA and nascent DNA. ( b , c ) Inhibition of UTX activity by GSK J4 ( b ) and CBP activity by C646 ( c ) leads to early accumulation of H3K27me3 (left) and loss of H3K27ac (right). Embryos were incubated with (left columns) or without (right columns) GSK J4 ( b ) or C646 ( c ). They were then labelled with EdU for 15 min, followed by the PLA between biotin and either H3K27me3 or H3K27ac. Following CAA, embryos were immunostained for biotin (EdU, in green). ( d ) A scheme of proposed inhibition of H3K27 methylation by E(z) by CBP and UTX following DNA replication. The results are from four independent experiments. Scale bar, 10 μm. Full size image Demethylation by UTX may not be the only mechanism causing a delay in H3K27 methylation after DNA replication. Importantly, the Drosophila HAT CBP acetylates histone H3 at K27, and thus antagonizes methylation of the same residue by E(z) [18] . Thus, in addition to demethylation of K27me3 by UTX, proximity of CBP to DNA during replication may provides an additional mechanism in which acetylation of H3K27 may preclude methylation of H3K27 by E(z). Drosophila CBP is in close proximity to PCNA and nascent DNA labelled from 5 min to 2 h ( Fig. 3b ). CBP associates with TRX in the TAC1 complex [19] , and also forms a complex with UTX [20] . Both TRX [4] and UTX ( Fig. 3a ) are associated with DNA after 5 min of EdU labelling, suggesting that CBP may be present on nascent DNA in two distinct protein complexes. H3K27ac is detectable on nascent DNA at 10 min after DNA replication ( Fig. 3c ). Inhibition of CBP activity with the C646 inhibitor leads to a significant decrease in H3K27ac 15 min after DNA replication ( Fig. 3g ), and as a potential consequence to the emergence of H3K27me3 ( Fig. 3f ). We also detected a loss of H3K27ac in embryos treated with UTX inhibitor ( Fig. 3e ), which is consistent with the proposed role of UTX in CBP activity [20] . In summary, our results indicate that both acetylation of H3K27 by CBP and demethylation of H3K27 by UTX may prevent accumulation of H3K27me3 at early stages following DNA replication (scheme in Fig. 3h ). It is possible that upregulation of the activity of E(z) and/or diminishing activities of CBP and UTX contribute to accumulation of H3K27me3 at the completion of the S phase [4] . At this time (1 and 2 h of EdU labelling), the presence of both H3K27ac and H3K27me3 ( Fig. 3c , Table 1 and (ref. 4 )) likely reflects the accumulation of these histone forms in different regions of the genome. HP1 may be an epigenetic mark of heterochromatin The combination of PLA and CAA assays also allows us to test the order of recruitment of heterochromatic proteins in the S phase. Methylation of H3K9 by Clr4, a Schizosaccharomyces pombe homologue of the Drosophila Su(Var)3–9, was proposed to create an epigenetic mark that is recognized by the chromo domain of the heterochromatin protein 1 (HP1) that mediates gene silencing [21] , providing a stepwise model for formation of the transcriptionally silent heterochromatin. Another model [22] suggests that HP1 is recruited to replication forks through direct interaction with histone chaperone CAF1 (ref. 23 ) that is associated with PCNA. HP1 then recruits SUV39H that induces the full extent of methylation of H3K9. According to this model, H3K9me3 may be transferred to daughter strands, although its role as an epigenetic mark is not clear. We show that HP1 is in proximity to PCNA and with short nascent DNA ( Fig. 4a ). In contrast, Su(Var)3–9 is not found in proximity to PCNA, but is found on nascent DNA in 5 min after DNA replication ( Fig. 4b ). H3K9me3 is detected shortly after recruitment of this enzyme at 10 min after DNA replication ( Fig. 4c ). On the basis of these results, we propose a new order of assembly of heterochromatin in Drosophila ( Fig. 4d ). HP1, but not H3K9me3, may serve as an epigenetic mark during DNA replication. As Su(Var)3–9 and HP1 interact and are interdependent in their localization in Drosophila heterochromatin [24] , it is possible that HP1 recruits Su(Var)3–9 shortly after the passage of the replication fork. Association of Su(Var)3–9 may lead to fast methylation of H3K9, finalizing the formation of the heterochromatin. Our results do not rule out the possibility that parental H3K9me3 is demethylated, transferred to nascent DNA and is methylated at K9 after Su(Var)3–9 is recruited. 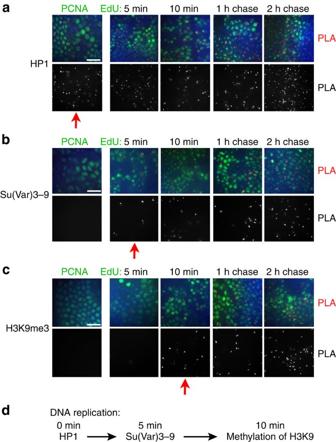Figure 4: Heterochromatin proteins are found in proximity to nascent DNA in defined order following replication. Antibodies againstDrosophilaHP1 protein (a), H3K9 histone methyltransferase Su(Var)3–9 (b) and H3K9me3 (c) were used for PLA with PCNA (left column) and for CAA with EdU-labelled DNA (columns 2–5). Red arrows indicate when proteins are first detected in these experiments. A scheme of proposed sequence of formation of heterochromatin is shown ind. The results are from three independent experiments. Scale bar, 10 μm. Figure 4: Heterochromatin proteins are found in proximity to nascent DNA in defined order following replication. Antibodies against Drosophila HP1 protein ( a ), H3K9 histone methyltransferase Su(Var)3–9 ( b ) and H3K9me3 ( c ) were used for PLA with PCNA (left column) and for CAA with EdU-labelled DNA (columns 2–5). Red arrows indicate when proteins are first detected in these experiments. A scheme of proposed sequence of formation of heterochromatin is shown in d . The results are from three independent experiments. Scale bar, 10 μm. Full size image Arginine methyltransferases are in proximity to nascent DNA To expand our analysis of chromatin proteins that associate with nascent DNA, we examined PRMT arginine methyltransferases that methylate numerous proteins including histones. Although their epigenetic role is not well defined, their ability to methylate histones may potentially impact the epigenetic state of the gene [25] , [26] . Drosophila DART1 and DART4 are arginine methyltransferases (homologous to mammalian PRMT1 and PRMT4/CARM1, respectively) that catalyse formation of the assymetrical dimethylated arginine residues in histones H4 and H3 (ref. 27 ). Similar to lysine methyltransferases, DART1 and DART4 are found in proximity to PCNA and nascent DNA labelled with EdU for 5 min ( Fig. 5a,b and Table 1 ). Interestingly, H3R17me2 and H4R3me2, two products of these enzymes, are not associated with PCNA and are detected at nascent DNA at different times following DNA replication ( Fig. 5c,d and Table 1 ). In addition, pCAF, another Drosophila HAT protein, the histone deacetylase HDAC1 and the PcG DNA-binding protein PHO are all in proximity to PCNA and nascent DNA labelled from 5 min to 2 h ( Figure 6 and Table 1 ). 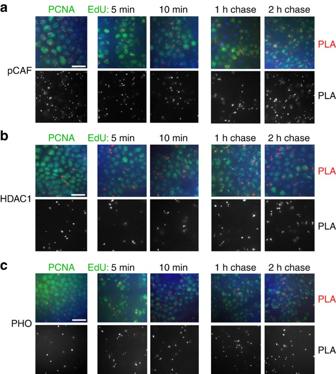Figure 6: pCAF and HDAC1 and PHO are in proximity to PCNA and nascent DNA. Antibodies againstDrosophilapCAF (a), HDAC1 (b) and PHO (c) were used for PLA with PCNA (left column) and for CAA with EdU-labelled DNA (columns 2–5). The results are from three independent experiments. Scale bar, 10 μm. 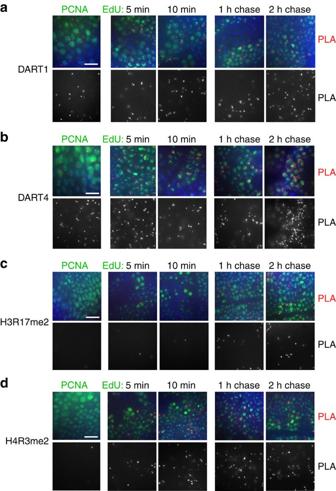In summary, most tested histone modifiers, chromosomal and DNA-binding proteins are found in close proximity to PCNA and nascent DNA shortly after replication. Figure 5: Proximity of arginine methyltransferases and their products to PCNA and nascent DNA. (a,b) DART1 and DART4 are in proximity to PCNA and nascent DNA. Antibodies againstDrosophilaDART1 and DART4 were used for PLA with PCNA (left column) and for CAA with EdU-labelled DNA (columns 2–5). (c,d) Histones are methylated at arginines following DNA replication. Antibodies against H3R17me2a and H4R3me2a were used for PLA with PCNA (left column) and for CAA with EdU-labelled DNA (columns 2–5). The results are from three independent experiments. Scale bar, 10 μm. Figure 5: Proximity of arginine methyltransferases and their products to PCNA and nascent DNA. ( a , b ) DART1 and DART4 are in proximity to PCNA and nascent DNA. Antibodies against Drosophila DART1 and DART4 were used for PLA with PCNA (left column) and for CAA with EdU-labelled DNA (columns 2–5). ( c , d ) Histones are methylated at arginines following DNA replication. Antibodies against H3R17me2a and H4R3me2a were used for PLA with PCNA (left column) and for CAA with EdU-labelled DNA (columns 2–5). The results are from three independent experiments. Scale bar, 10 μm. Full size image Figure 6: pCAF and HDAC1 and PHO are in proximity to PCNA and nascent DNA. Antibodies against Drosophila pCAF ( a ), HDAC1 ( b ) and PHO ( c ) were used for PLA with PCNA (left column) and for CAA with EdU-labelled DNA (columns 2–5). The results are from three independent experiments. Scale bar, 10 μm. Full size image Chromatin remodelers are dissociated during DNA replication Chromatin-remodelling complexes are essential for gene regulation [28] , [29] , hence we examined the behaviour of subunits of chromatin-remodelling complexes during DNA replication. ISWI is the catalytic subunit of several distinct ATP-dependent chromatin-remodelling complexes that have essential roles in regulation of higher-order chromatin structure [30] , [31] , [32] . Unlike most of chromatin-modifying enzymes examined above, ISWI is not in proximity to PCNA and appears on nascent DNA only after 10 min of DNA replication ( Fig. 7a ). The Drosophila TrxG protein BRM is an ATPase [33] present in two distinct complexes, BAP and PBAP. These complexes share seven identical subunits. The TrxG protein OSA is a component of BAP but not PBAP [34] . In contrast, Polybromo is a component of PBAP but not BAP [35] . Neither BRM nor OSA nor Polybromo are in proximity to PCNA, and they are not found at nascent DNA labelled with EdU for 5 min ( Fig. 7b–d ). Interestingly, although BRM and Polybromo are first detected on nascent DNA at 10 min, OSA is not detected until 2 h of EdU incorporation ( Fig. 7b–d ). These results suggest that, although both BAP and PBAP complexes dissociate from DNA during replication, these distinct chromatin-remodelling complexes are recruited to their sites on DNA at significantly different times following DNA replication. As the four tested proteins are components of many major chromatin-remodelling complexes ( Table 1 ), our results suggest that chromosomal-remodelling complexes are dissociated from DNA for longer periods than most histone-modifying complexes. 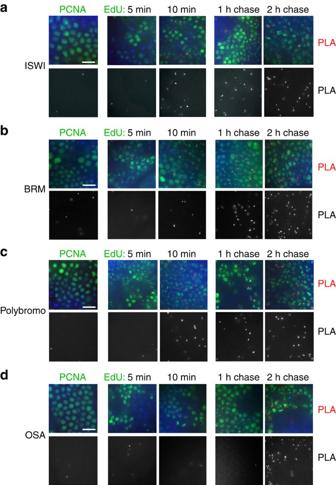Figure 7: Recruitment of chromatin remodeling proteins to nascent DNA. Antibodies againstDrosophilachromatin remodelers ISWI (a), BRM (b), Polybromo (c) and OSA (d) were used for PLA with PCNA (left column) and for CAA with EdU-labelled DNA (columns 2–5). ISWI, BRM and Polybromo are first detected on DNA labelled with EdU for 10 min. OSA is first detected on DNA labelled for 2 h. The results are from three independent experiments. Scale bar, 10 μm. Figure 7: Recruitment of chromatin remodeling proteins to nascent DNA. Antibodies against Drosophila chromatin remodelers ISWI ( a ), BRM ( b ), Polybromo ( c ) and OSA ( d ) were used for PLA with PCNA (left column) and for CAA with EdU-labelled DNA (columns 2–5). ISWI, BRM and Polybromo are first detected on DNA labelled with EdU for 10 min. OSA is first detected on DNA labelled for 2 h. The results are from three independent experiments. Scale bar, 10 μm. Full size image Interestingly, a CBP complex with UTX also includes BRM [20] . Our results suggest that only two components of this complex, UTX and CBP, are in proximity to PCNA and nascent DNA labelled for 5 min with EdU, whereas BRM is associated with nascent DNA only after 10 min of EdU labelling ( Figs 3a,b and 7b ). This suggests that the BRM component of the triple UTX–CBP–BRM complex is dissociated from this complex during replication. Thus, during replication CBP may exist in two complexes, with TRX and with UTX, and the BRM component of the UTX–CBP complex is recruited later after DNA replication. This study examines the recruitment of multiple proteins to daughter DNA following DNA replication in vivo . The surprising finding of this work is that with the exceptions of ASH1 and Su(Var)3–9, many histone-modifying proteins that belong to several different functional groups are found in close proximity to PCNA and short nascent DNA. It is likely that these proteins may be transiently dissociated and kept in the vicinity of the replication fork through interactions with PCNA or other replication proteins, and are then rapidly recruited to nascent DNA. It is also possible, that similar to PcG proteins, some of chromatin proteins remain associated with DNA during replication [5] , [6] . Our results suggest that modifications of histones on daughter DNA occur later after replication, and may be governed by complex activities of histone-modifying proteins associated with nascent DNA. We suggest that histone methylation by itself is unlikely to be an epigenetic mark [36] . Instead, we propose that many chromatin proteins are required early after DNA replication to re-establish transcriptional states. The methods applied here allow examination of the order of assembly of chromatin. This essential step forward allowed us to examine previously proposed models of epigenetic marking and stepwise assembly of chromatin. In particular, we found that HP1 has an essential early role in formation of heterochromatin. The timing of appearance of other key players suggests that Su(Var)3–9 may be recruited by HP1, and that methylation of H3K9 by this protein occurs shortly afterwards. These results agree with previous studies that demonstrated physical interactions between HP1 and Su(Var)3–9. Our studies establish the exact order of events following DNA replication in Drosophila embryos, but do not describe the molecular mechanisms. This work ( Table 1 ) and our previous data [4] show that unlike histone modifiers, modified histones are accumulated at different times after DNA replication. With the exception of the H4K5ac mark associated with newly synthesized histones, we are unable to determine whether parental, newly synthesized histones or both are acquiring modifications in our experiments. Our data suggest that the histone modification is temporally regulated. Using CAA, it is now possible to functionally assess the roles of histone-modifying enzymes in temporal regulation of histone modification. In particular, we found that methylation of H3 at K27 by E(z), a hallmark of repressed genes in euchromatin, is delayed due to the activities of HAT CBP and de-HMT UTX. The antagonistic effects of these modifiers were described previously [18] , [20] . Importantly, our work places them in the context of the cell cycle and in the gradual maturation of chromatin following DNA replication. An important result of this work is that unlike histone-modifying proteins, members of several nucleosome-remodelling complexes dissociate from DNA and re-associate with nascent DNA at different times, perhaps after the end of the S phase, or are developmentally regulated. The mechanisms of recruitment of these proteins following DNA replication are not known. Chromatin remodelers are thought to be recruited to their target genes by transcription factors and modified histones, in particular acetylated nucleosomal histones [37] , [38] . The results of this and our previous work suggest that modified histones tested so far are detected on nascent DNA with various delays [4] ( Table 1 ). Thus, one explanation of the late recruitment of chromatin remodelers may stem from delays in accumulation of histone modifications that are essential to recruit these proteins. Significantly, these results suggest that chromatin remodelers do not have direct roles in maintaining epigenetic information during replication and that their roles in transcription may be significantly delayed compared with that of histone-modifying complexes. Overall, the results of this work demonstrate that in early Drosophila embryos the structure of chromatin may be disrupted for only very short time by DNA replication, and that modification of histones may be a complex orderly process that follows DNA replication. They also suggest that histone modification is unlikely to be an early event in chromatin assembly on nascent DNA or to have a causal role in assembly of specific chromatin environments. We propose that epigenetic marking during replication may require many proteins to be present soon after replication to reconstitute the chromatin environment. PLA assays Embryos were dechorionated in 50% bleach and fixed in a 1:1 mixture of 4% formaldehyde in PBS and heptane for 20 min, washed, blocked and incubated overnight at 4 °C with primary antibodies from different species. PLA assays (Olink Bioscience) were performed as follows: secondary antibodies with conjugated oligonucleotides (MINUS and PLUS probes) were incubated for 1 h at 37 °C (ref. 4 ). Two oligonucleotides that hybridize to the two PLA probes were added and ligated with DNA ligase for 30 min at 37 °C. A closed circle forms if proteins are in close proximity. PCR rolling circle amplification by polymerase was carried out in the presence of fluorescent-labelled oligonucleotides for 100 min in the dark at 37 °C. Following PLA reactions, PCNA or EdU were detected in embryos by incubation with FITC-conjugated anti-mouse antibody. In vivo CAAs Nascent DNA was labelled with 250 μM of EdU in Drosophila Schneider Medium for 5, 10 and a 10 min pulse followed by chase for 1 and 2 h. Embryos were fixed in 4% formaldehyde in PBS for 20 min. Following incorporation of EdU and fixation, embryos were subjected to Click-iT reaction (Invitrogen) for 30 min in the dark to add biotin to the EdU. Embryos were washed, blocked in the blocking buffer for antibody incubation (Roche) and incubated with mouse monoclonal anti-biotin antibody and the rabbit antibody of interest at 4 °C overnight as described [4] . The PLA reaction was performed as described above. Following PLA, EdU was detected by incubation with FITC-conjugated anti-mouse antibody. In experiments using inhibitors, embryos were incubated in the Drosophila Schneider Medium with 40 μM of the CBP inhibitor C646 (Sigma) for 1 h or with 100 μM of the UTX inhibitor GSK J4 (Tocris Bioscience) for 1 h 30 min that were dissolved in DMSO. In control experiments, embryos were incubated for the same time with the same concentration of DMSO but without inhibitors. Embryos were then labelled with EdU for 15 min. CAA was performed with antibodies against H3K4me3 and H3K27ac. Nucleus to nucleus variability in the CAA assays is large. Several reasons may contribute to this variability. Different nuclei in the embryo are at different stages in the S phase, hence there is variation in the relative amounts of euchromatin and heterochromatin being replicated in particular embryos. It is possible that variability of permeabilization of embryos during 5–10 min labelling with EdU causes some inconsistencies. Embryos are three dimensional, and depending on the Z plane, different amounts of the peripheral versus central nucleus can be present, thus altering the number of detectable signals. Antibodies The following antibodies were used: H3K4me1 (1:2,000, Active Motif); H3K4me2 (1:2,000, Active Motif); H3K9me3 (1:2,000, Active Motif); H3R17me2 (1:2,000, Active Motif); H4R3me2 (1:4,000, Active Motif); PCNA (1:5,000, Abcam); ASH1 (ref. 39 ) (1:1,000); dSET1 (ref. 10 ) (1:500); LID [15] (1:1,000); LSD [12] (1:3,000); PHO [40] (1:2,000); UTX [16] (1:1,000), DART1 and DART4 (ref. 27 ) (1:1,000 and 1:2,000, respectively); CBP and pCAF [19] (1:2,500 and 1:2,000, respectively); HDAC1 (1:2,000, Abcam); BRM [33] (1:500); OSA and HP1 (1:3,000 and 1:5,000, respectively, Developmental Hybridoma Bank); ISWI (1:2,000, Abcam); H3K27Ac (1:2,000, Active Motif); Polybromo [35] (1:2,000); Su(Var)3–9 (1:300, Abcam). Examination of embryos Drosophila wild-type strain Oregon R embryos were examined from gastrulation to mid-embryogenesis (4–6 h after egg lay, AEL). All antibodies used in this study detect nuclear localization of all examined proteins. The concentrations of all antibodies were adjusted by immunofluorescence to minimize potential non-specific interactions before their use in PLA and CAA assays. Specificity controls included PLA reactions with only one antibody. None of the antibodies used showed any significant number of PLA signals in these control experiments. Specificity of PLA was monitored by examining whether PLA signals are detected only in the PCNA- and EdU-labelled nuclei. PLA signals were counted in 300–400 nuclei from several embryos in at least three independent experiments. Figure images reflect the results of a typical experiment. The assessment of the numbers of PLA signals in Table 1 is explained in the legend to Table 1 . Western blotting A quantity of 0.25 mg of nuclear extract prepared from Drosophila embryos was immunoprecipitated with PCNA antibody or with IgG as a negative control. The immunoprecipitated material was analysed by western blotting with antibodies against Polycomb and Trithorax. How to cite this article: Petruk, S. et al. Stepwise histone modifications are mediated by multiple enzymes that rapidly associate with nascent DNA during replication. Nat. Commun. 4:2841 doi: 10.1038/ncomms3841 (2013).